Robust and versatile ionic liquid microarrays achieved by microcontact printing Lab-on-a-chip and miniaturized systems have gained significant popularity motivated by marked differences in material performance at the micro-to-nano-scale realm. However, to fully exploit micro-to-nano-scale chemistry, solvent volatility and lack of reproducibility need to be overcome. Here, we combine the non-volatile and versatile nature of ionic liquids with microcontact printing in an attempt to establish a facile protocol for high throughput fabrication of open microreactors and microfluidics. The micropatterned ionic liquid droplets have been demonstrated as electrochemical cells and reactors for microfabrication of metals and charge transfer complexes, substrates for immobilization of proteins and as membrane-free high-performance amperometric gas sensor arrays. The results suggest that miniaturized ionic liquid systems can be used to solve the problems of solvent volatility and slow mass transport in viscous ionic liquids in lab-on-a-chip devices, thus providing a versatile platform for a diverse number of applications. Increasing attention has been given to device-miniaturization technology over the past decades owing to its significant advantages for macro/lab-scale chemistry, such as material conservation, fast response or reaction time and high product yield [1] , [2] , [3] . In addition, some violent reactions that are not feasible to be carried out on macroscale can be performed using lab-on-a-chip [1] . Nevertheless, device-miniaturization technologies face several challenges, of which solvent evaporation is one of the major issues [2] . Fast evaporation of volatile organic solvents in open microsystems is responsible for variation in solvent volume and change in concentration of components with time, resulting in unreliable products or analytical results. Furthermore, traditional organic solvents are prone to vapour cross-contamination, which might even cause the device to stop functioning properly [3] . Several approaches have been proposed to circumvent this issue, such as containing the solvent within channels or ‘walls’, which, however, are difficult to miniaturize and can suffer from problems such as large dead volume, obstruction of channels and poor control of hydrodynamic pressure [2] , [4] . Another suggested solution is to create an on-chip solvent reservoir in order to keep up with the evaporative losses [5] . This technique is also haunted with problems such as the large amount of space required for solvent storage, and is impractical for devices with multiple solvents [3] . The absence of standard apparatus forces most labs to develop their own custom components, which in turn makes such a device a one-of-a-kind with very little diversity or reproducibility [5] . An alternative approach adopted here to address the issue is to use solvents that are non-volatile allowing fabrication of open micropatterns and microreactor systems, also called a ‘wall-less’ design. Ionic liquids (ILs) are a class of solvents with good thermal and chemical stability that typically have negligible vapour pressure [6] . They have demonstrated applications in almost every field of chemistry, ranging from electrochemistry, organic synthesis to biological applications [6] . The values of non-volatile ILs in microsystems have been appreciated in several early studies. For example, Hozumi et al. [7] have utilized ILs in photolithography as a medium for smart visualization of submicron-scale structures. Huang et al. [8] applied ILs as electrolytes and developed a membrane-free amperometric gas sensor which can operate in extreme conditions such as high temperature and pressure. Dubois et al. [2] have fabricated IL droplets (300 nl) on a chip surface using Eppendorf micropipettes, and they demonstrated that efficient organic synthesis can be achieved inside the stable IL-droplet reactors [9] . Very recently, Jeong et al. [10] applied a small drop of IL (100 nl) as electrolyte to convert a metal oxide (VO 2 ) from an insulating to a conducting state, demonstrating the enormous potential of using non-volatile IL droplets for fabrication of non-volatile memory and logic chips. Fostered by diverse applications of ILs and lab-on-a-chip devices, it is desirable to develop microfabrication protocols for IL-based miniature devices with high reproducibility and high throughput. Herein we report a facile and reproducible approach for fabrication of IL patterns using microcontact printing (μCP), and report its use in the development of a gas sensor. μCP is a popular microfabrication method that can generate patterns with molecular-level detail, high fidelity, low cost and high scalability [11] . However, μCP methodology for ILs has not been established so far. In this study, we combine μCP with ILs and fabricate a series of IL micropatterns on gold and glass substrates. Several printing strategies have been established and tailored to ILs used in specific applications. We demonstrate that microfabrication of IL micropatterns gives versatile platforms for a range of applications. μCP of IL s A standard μCP method is applied to transfer 11-mercaptoundecanoic acid (MUA) onto a gold-coated glass slide to form hydrophilic zones as a result of the terminal –COOH groups. Gaps are refilled with hexadecanethiol (HDT) to form hydrophobic, CH 3 -terminated zones ( Supplementary Fig. 1 ) [11] . A drop of air-equilibrated IL (for example, 1-butyl-3-methyl immidazolium tetrafluoroborate, [BMIM][BF 4 ]) is brought into contact with the printed area for 1–2 s and excessive IL is removed by back suction. IL selectively attaches to the hydrophilic zones and forms arrays of IL droplets with uniform shape and size throughout the entire printed area that is shown in Fig. 1a–c . Detailed investigation on microdroplets shows that a very thin film of IL is formed on the microstructures with clear straight edges ( Fig. 1b ), attributed to the well-defined surface chemistry of the underlying self-assembled monolayers (SAMs). The film thickness in the middle of the droplet was measured as 9±1 μm by scanning confocal microscopy. A range of ILs including aprotic ILs (for example, [BMIM][BF 4 ] and [BMIM][PF 6 ]) and protic ILs (for example, ethylammonium nitrate, ethylammonium nitrate (EAN) and triethylammonium methylsulphonate (TAMS)) with distinctly different hydrophobicity, viscosity and acidity have been applied and each forms good quality patterns. It is noteworthy that, regardless of the hydrophobicity of the ILs (for example, [BMIM][BF 4 ] is hydrophilic and [BMIM][PF 6 ] is hydrophobic), they all adsorb preferentially to regions of MUA. This is attributed to different strengths of intermolecular forces between two surfaces, which generally follow a trend of hydrophilic/hydrophilic>hydrophilic/hydrophobic>hydrophobic/hydrophobic [12] , and so even a hydrophobic IL will bond to the hydrophilic surface in preference to the hydrophobic areas. The approach can be easily adapted for fabrication of more complex two-dimensional microstructures ( Supplementary Fig. 2a ), which are useful for applications requiring microreactors and microfluidics. 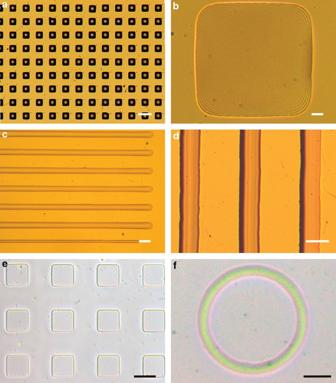Figure 1: Images of ionic liquid micropatterns. (a–d) Reflection micrographs of micropatterns of [BMIM][BF4] fabricated on a gold surface via (a–c) indirect printing (scale bar, 100 μm (a), 10 μm (b) and 100 μm (c)) and (d) partial printing (scale bar, 30 μm); (e,f) Phase contrast micrographs of micropatterns of a protic IL [EDA][acetate] fabricated on a glass surface via direct printing (scale bar, 50 μm (e) and 25 μm (f)). Figure 1: Images of ionic liquid micropatterns. ( a – d ) Reflection micrographs of micropatterns of [BMIM][BF 4 ] fabricated on a gold surface via ( a – c ) indirect printing (scale bar, 100 μm ( a ), 10 μm ( b ) and 100 μm ( c )) and ( d ) partial printing (scale bar, 30 μm); ( e , f ) Phase contrast micrographs of micropatterns of a protic IL [EDA][acetate] fabricated on a glass surface via direct printing (scale bar, 50 μm ( e ) and 25 μm ( f )). Full size image Applying an IL onto a gold surface patterned with HDT SAMs, without filling the gap with MUA, also results in stable IL micropatterns ( Fig. 1d ). The IL droplet formed via this ‘partial printing’ strategy ( Supplementary Fig. 3 ) is in direct contact with the bare gold surface and could be used as open micro-electrochemical cells. It is also possible to form an IL array by directly using an IL as the ink. However, IL patterns formed via this approach are generally less uniform in size and shape ( Supplementary Fig. 2b ), and mechanically unstable owing to the weak interaction between an IL and the bare gold surface. To enhance the interaction between an IL and a gold substrate, we developed a ‘semi-direct’ approach by dissolving a thiol into the IL to be printed ( Supplementary Fig. 4 ), and hypothesizing the formation of thiol–gold bonds, and then IL–thiol interactions will help to anchor the ILs onto the surface and enhance the stability of IL patterns. Previous studies also have used ILs as solvents for dissolution of thiols, and showed that structurally more stable SAMs can be formed on a gold surface [13] . 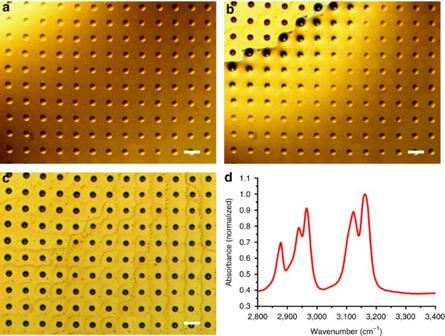Figure 2: Stable ionic liquid microarray immersed in a nonpolar solvent. (a–c) Reflection micrographs of [BMIM][BF4] on a gold surface when submerged in hexane (scale bar, 100 μm) (a), during evaporation (scale bar, 100 μm) (b) and after the complete evaporation of hexane (scale bar, 100 μm) (c); (d) Fourier transform infrared spectra recorded from a droplet in (c) confirming that the droplet is [BMIM][BF4]. Supplementary Figure 2c shows micropatterns of [BMIM][PF 6 ] containing dissolved MUA fabricated by the ‘semi-direct’ approach. The patterns formed by this approach are more uniform and physically more stable compared with those obtained through ‘direct printing’. The ‘semi-direct’ printing results give us the confidence that ‘direct printing’ of ILs is possible if strong IL-surface interactions or bonding can be established. To demonstrate that ‘direct printing’ of ILs is achievable, and also that ILs can be printed onto substrates other than gold, two protic ILs, ethylenediammonium acetate (EDAA) and ethylenediammonium formate (EDAF), were prepared according to the method described previously [14] and applied as ink for direct printing onto glass ( Supplementary Fig. 5 ). The EDA cation in each IL contains two amine groups. A microscopic glass slide was pre-coated with –COOH-terminated SAMs by treatment with phosphonohexadecanoic acid (PHDA) [15] . Figure 1e,f shows that well-defined, mechanically stable IL micropatterns are obtained on glass substrates by amine–carboxylic acid cross-linking [16] . It is noteworthy that ILs are ‘designable’ solvents and can be functionalized with specific groups for specific tasks such as thiol-functionalized ILs for attachment onto the gold surface [17] . We anticipate that direct printing can be particularly useful for micropatterning of task-specific ILs by employing a range of surface cross-linking chemistry [16] . Characterization of IL micropatterns We estimate the volume of IL in a single microdroplet. Typically, for a 50 μm diameter circular droplet, assuming a spherical cap shape and a height of 10 μm in the centre, the volume is calculated to be 9.2 pl, which corresponds to a surface-to-volume ratio of 2.4 × 10 3 cm 2 l −1 . This volume is >5 orders of magnitude smaller than that can normally be prepared by using a micropipette [2] . The small volume and large surface-to-volume ratio are not only advantageous for conserving ILs, which are relatively costly materials, but also for a number of gas adsorption-based applications such as gas sensing or CO 2 capture [18] , [19] . Further reduction in droplet volume can be achieved by decreasing the size of microstructures and/or using spin coating to achieve thinner IL droplets ( Supplementary Fig. 2d ). [BMIM][BF 4 ] micropatterns obtained by ‘indirect printing’ show excellent mechanical stability in air (they survive when sample slides are tilted, turned upside down or even thrown from a height) and thermal stability up to 50 °C. Intriguingly, hydrophilic [BMIM][BF 4 ] microdroplets are found to be stable when immersed into a range of nonpolar solvents. Figure 2 shows that [BMIM][BF 4 ] micropatterns remain unchanged when repetitively immersed in hexane. Infrared (IR) spectra recorded on the microdroplet before and after immersion into hexane are indistinguishable, showing characteristic bands of [BMIM][BF 4 ] at 2,878, 2,940, 2,966, 3,122 and 3,162 cm −1 , respectively [20] . These liquid-stable IL microdroplets may find applications in understanding the fundamental properties of micro-scale interfaces between immiscible liquids, as well as a range of applications at liquid–liquid interfaces such as electrochemical sensors, solvent extraction, pharmacokinetics and solar energy conversion [21] . Figure 2: Stable ionic liquid microarray immersed in a nonpolar solvent. ( a – c ) Reflection micrographs of [BMIM][BF 4 ] on a gold surface when submerged in hexane (scale bar, 100 μm) ( a ), during evaporation (scale bar, 100 μm) ( b ) and after the complete evaporation of hexane (scale bar, 100 μm) ( c ); ( d ) Fourier transform infrared spectra recorded from a droplet in ( c ) confirming that the droplet is [BMIM][BF 4 ]. Full size image Metal electrodeposition from IL micropatterns The micropatterned IL droplets provide a versatile platform for a range of applications. We demonstrate first the application of IL droplets as open electrochemical cells for microelectrodeposition of technologically important metals such as Ag and Cu ( Supplementary Fig. 6 ) [22] , [23] , [24] , [25] . A protic IL (for example, EAN and TAMS) containing dissolved Ag + or Cu 2+ is patterned on a gold substrate via the ‘partial printing’ method. Protic ILs are chosen because of the high solubilities of Ag + and Cu 2+ [24] , [25] . Cyclic voltammograms were recorded at a gold electrode to identify the electrodeposition potentials ( E dep ) ( Supplementary Fig. 7 ). Controlled potential deposition of Ag was then carried out at E dep =−0.1 V versus Ag quasi-reference electrode (QRE) for 60 s, to form well-defined silver micropatterns, as confirmed with scanning electron microscopy (SEM) and energy dispersive X-ray (EDX) analysis ( Fig. 3a ; Supplementary Fig. 8 ). Electrodeposition of Cu performed at E dep =−0.2 V versus Cu QRE for 60 s also leads to formation of a Cu micropattern on gold ( Supplementary Figs 9 and 10 ). These experiments prove the concept of using micropatterned IL droplets as templated electrochemical cells for fabrication of metal microstructures on a surface, which could potentially be used for fabrication of integrated circuits and interconnects. 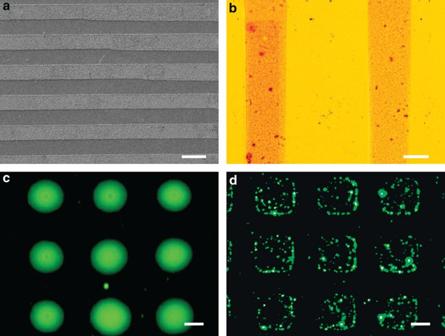Figure 3: Applications of ionic liquid micropatterns. (a) SEM micrograph of silver patterns electrodeposited onto a gold substrate from microprinted EAN containing 1 M Ag+(scale bar, 100 μm); (b) micrograph of AgTCNQ electrodeposited from micropatterned [BMIM][BF4] from 3.33 mM Ag+and 3.33 mM TCNQ for 300 s (scale bar, 25 μm); (c,d) fluorescence micrographs of micropatterned [BMIM][BF4] containing dissolved (c) 10 μM Cytc-OG488 (scale bar, 25 μm) and (d) 0.753 μM BSA–FITC (scale bar, 25 μm), respectively. Figure 3: Applications of ionic liquid micropatterns. ( a ) SEM micrograph of silver patterns electrodeposited onto a gold substrate from microprinted EAN containing 1 M Ag + (scale bar, 100 μm); ( b ) micrograph of AgTCNQ electrodeposited from micropatterned [BMIM][BF 4 ] from 3.33 mM Ag + and 3.33 mM TCNQ for 300 s (scale bar, 25 μm); ( c , d ) fluorescence micrographs of micropatterned [BMIM][BF 4 ] containing dissolved ( c ) 10 μM Cyt c -OG488 (scale bar, 25 μm) and ( d ) 0.753 μM BSA–FITC (scale bar, 25 μm), respectively. Full size image Microfabrication of charge-transfer complexes AgTCNQ We further demonstrate the utilization of the IL microdroplets for fabrication of charge-transfer complexes of silver tetracyanoquinodimethane (AgTCNQ), an attractive organic semiconductor for non-volatile memory because of its reproducible nanosecond electrical and optical switching behaviour and memory effects [23] , [26] . AgTCNQ can be fabricated via two routes from IL microdroplets. The first ‘electrocrystallization’ route employs open [BMIM][BF 4 ] micro-electrochemical cells containing equimolar (3.33 mM) Ag + and TCNQ [23] . Controlled potential crystallization at −0.8 V for 300 s forms AgTCNQ by the spontaneous reaction between dissolved TCNQ and the electrodeposited Ag metal ( Supplementary Fig. 11 ). AgTCNQ micropatterns were examined by SEM ( Fig. 3b ). EDX analysis reveal electrocrystallized materials containing Ag, C and N, as expected for AgTCNQ formation [23] . In the second route, AgTCNQ is fabricated by photocrystallization [26] , using the IL microdroplets as photoreactors ( Supplementary Fig. 12 ). In this approach, [BMIM][BF 4 ] containing equimolar (3.33 mM) Ag + and TCNQ and 10% volume fraction benzyl alcohol as a sacrificial electron donor was patterned onto a gold surface via ‘indirect printing’. Irradiating the IL patterns at λ =425 nm for 5 min led to the detection of visible colour change of the IL-patterned zone from yellow to blue, and then dark blue with extended irradiation times. This is consistent with previous observations [26] , and is attributed to the photoreduction of TCNQ to TCNQ − radical anions, which react with Ag + forming dark blue AgTCNQ crystals, as confirmed by microscopy investigation ( Supplementary Fig. 13 ). These data show the promise of using an array of IL microdroplets as photoreactors for screening a range of photochemical reactions in ILs [26] , [27] . Protein micropatterning using ILs as immobilization media ILs have demonstrated considerable applications for biocatalysis, biotransformations, protein-based pharmaceutical preparations and cellular therapies [28] . While many ILs are not biocompatible, some have been shown to be useful media for solubilization, immobilization and stabilization of biological molecules such as enzymes, DNA and proteins with retained activities [29] . These ILs can thus be used for micropatterning of biomolecules that have high stability by simply dissolving in the ILs and then printing as microdroplets onto a surface. Figure 3c illustrates the fabrication of protein microarrays of cytochrome c (Cyt c ), a highly studied redox protein, which can be solubilized and remain active even in dry ILs [30] . A 10-μM solution of Cyt c -OG488 (Oregon Green® 488) was prepared in [BMIM][BF 4 ] and then deposited on a gold chip patterned with 50 μm circles by ‘indirect printing’. Fluorescence images confirm the protein is patterned onto the surface and distributed evenly in the IL droplets. In another example, we patterned [BMIM][BF 4 ] containing dispersed bovine serum albumin/fluorescein isothiocyanate conjugate (BSA–FITC). The fluorescent images in Fig. 3d also show the immobilization of BSA within the IL droplets. Further study is under way to investigate the activity of proteins inside the IL droplets and to explore the use of these IL-based protein arrays for analytical/screening purposes. In addition, the versatility of ILs is such that their properties can be tailored to different biological reactions by mixing ILs with water, other ILs or organic solvents [29] , [31] all of which can be readily patterned using μCP ( Supplementary Fig. 14 ). Development of an amperometric microarray gas sensor Finally, we demonstrate a micropatterned IL interface as a unique platform for gas sensing. ILs have been regarded as ideal candidate electrolytes for replacing aqueous/organic solvent electrolytes in commercial gas sensors, which are prone to drying out and sensor failure, and for the development of membrane-free gas sensors ( Supplementary Fig. 15a,b ) [8] , [32] . However, current IL-based gas sensors suffer from one intrinsic drawback, namely the high viscosity of ILs [32] . The diffusion coefficients of gases (for example, O 2 ) in ILs are usually 1–2 orders of magnitude smaller than in aqueous or organic solvents [33] , [34] . This can significantly lower the sensitivity and response times of the sensors. Herein, we apply microcontact-printed IL droplets as a sensor for gaseous oxygen. Each IL microdroplet on the electrode serves as a sensing unit, forming a microarray gas sensor ( Supplementary Fig. 15c,d ). This sensor design benefits from the extremely small volume and thickness of each droplet, so diffusion distance is small and slow diffusion is not a significant issue. Furthermore, the extremely large surface-to-volume ratio, and high current density all help to improve the sensitivity, response time and overall quality of the signal from the sensors. 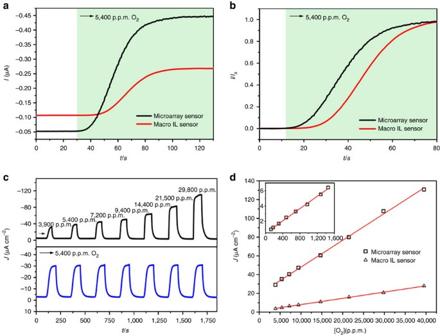Figure 4: Micropatterned IL droplets as amperometric gas sensor. (a) Amperometric current-time (I-t) and (b) normalized (I/Is) current-time responses of a IL microarray gas sensor versus a macrodisc electrode-based IL sensor, on exposure of 5,400 p.p.m. O2as indicated by the green background; (c) Current density-time (J-t) responses of a microarray sensor to different concentrations of O2(top) and replicate exposures to 5,400 p.p.m. O2(bottom); (d) calibration curves for a microarray sensor versus a macro-IL sensor. The inset is a calibration curve for a microarray sensor over a low concentration range (130–1,450 p.p.m.), where the macro-IL sensor shows no response. Figure 4a shows the amperometric current-time traces obtained at a [BMIM][NTf 2 ]-based microarray sensor in comparison with a conventional macroelectrode-based IL gas sensor for oxygen sensing. Lower background current is first observed for the microarray sensors, which is somewhat expected, as its electrode surface area is only ca. 1/3 of the macroelectrode. On the injection of O 2 (5,400 p.p.m., μl l −1 ), the current increases as O 2 is reduced at the applied potential (−1.2 V versus Ag). Remarkably, although the electrode surface area is smaller, the current obtained at the microarray sensor is significantly higher than the macroelectrode sensor. Taking into account the surface area, the current density obtained at the microarray sensor was found to be five times higher than the macro-IL sensor ( Supplementary Fig. 17 ). The high sensitivity could be attributed to the extremely large surface-to-volume ratio (fast gas adsorption) and small diffusion distance in each droplet. For better comparison of response time, the current response is further normalized by the plateau current ( I/Is ) ( Fig. 4b ) and the response times for the microarray sensor (25.1 s and 45.2 s to 50% and 90% of the plateau, respectively) are about 10 s faster than the macroelectrode sensor. The microarray sensor shows well-defined responses to different concentrations of O 2 and excellent reproducibility on exposure to constant O 2 concentration (5,400 p.p.m.) with a relative sample s.d. of 1.0% ( n =7, Fig. 4c ). The calibration curve shown for the microarray sensor in Fig. 4d exhibits excellent linearity over a wide concentration range of O 2 , and is significantly more sensitive than the macroelectrode sensor (curve slopes of 1 nA cm −2 per p.p.m. versus 0.07 nA cm −2 per p.p.m.) ( Table 1 ). The superior performance (for example, high sensitivity, fast response time and high reproducibility) of the microarray sensor is attributed to the much smaller and thinner IL droplets that can be prepared using μCP, which allows faster access of oxygen to the electrode surface despite the higher viscosity, and the non-volatile nature of ILs, as well as the mechanic stability of the IL micropatterns. It is worth noting that the membrane-free sensor design does not imply that the ILs will be exposed directly to an open atmosphere. A protective container such as a chamber or use of a filter will still be expected for the whole system design to prevent fouling by particulate contaminants. Figure 4: Micropatterned IL droplets as amperometric gas sensor. ( a ) Amperometric current-time ( I - t ) and ( b ) normalized ( I/I s ) current-time responses of a IL microarray gas sensor versus a macrodisc electrode-based IL sensor, on exposure of 5,400 p.p.m. O 2 as indicated by the green background; ( c ) Current density-time ( J - t ) responses of a microarray sensor to different concentrations of O 2 (top) and replicate exposures to 5,400 p.p.m. O 2 (bottom); ( d ) calibration curves for a microarray sensor versus a macro-IL sensor. The inset is a calibration curve for a microarray sensor over a low concentration range (130–1,450 p.p.m. ), where the macro-IL sensor shows no response. Full size image Table 1 Linear ranges, calibration equation, limit of detection (LOD) and limit of quantification (LOQ) for determination of O 2 using the IL microarray sensor. Full size table This work has established facile and reproducible protocols for micropatterning of ILs onto gold and glass surfaces. Several different printing strategies have been developed, namely indirect printing, partial printing, semi-direct printing and direct printing. These demonstrated the capability of the protocol to be customized for different ILs, substrate material in order to target specific applications. Characteristics of the fabricated micropatterns have been investigated by optical, physical and chemical methods, and we concluded that the IL micropatterns are very stable in air and even in some liquids. The excellent mechanical and thermal stabilities are important for commercial applications, including storage and transportation of these microchips. Micropatterned ILs are demonstrated in this study to be versatile for applications in microfabrication of metals and semiconductors via electrodeposition and photodeposition, and as media for protein immobilization to generate biological microarrays. Benefiting from a number of inherent advantages, including the non-volatility of ILs, their small volume, short diffusion distances to the surface for dissolved molecules and large surface-to-volume ratio, IL microarrays are demonstrated to be promising platforms for membrane-free gas sensors. In principle, analytical procedures or reactions that can be carried out in a macro-scale IL system can now be performed at the micro-scale level on a two-dimensional chip. The versatility of the IL microchips paves the way for a wide range of prospective functions that can be explored further for applications such as sensors, microreactor or microfluidic applications. Materials and chemicals High-purity 1-n-butyl-3-methylimidazolium tetrafluoroborate [BMIM][BF 4 ], 1-n-butyl-3-methylimidazolium bistriflimide [BMIM][NTf 2 ] and 1-n-butyl-3-methylimidazolium hexafluorophosphate [BMIM][PF 6 ] were purchased from Merck, ethylammonium nitrate (EAN) was purchased from Io-Li-Tec (>97%). Trichloromethyl silane 99%, 99% trichlorohexyl silane, ≥99% triethylamine, ≥99% ethylenediamine, 99% hexadecanethiol (HDT), 97% 11-mercaptoundecanoic acid (MUA), 97% 11-mercapto-1-hexanol (MOH), 99% 16-PHDA, 98% 7,7,8,8-tetracyanoquinodimethane (TCNQ), 99.99% silver tetrafluoroborate (AgBF 4 ) and bovine serum albumin-fluorescein isothiocyanate conjugate (BSA–FITC) were purchased from Sigma-Aldrich. Methane sulphonic acid 98%, and 99.99% copper nitrate (Cu(NO 3 ) 2 ) were purchased from Alfa Aesar. Milli-Q grade reagent water was used throughout the entire experiment for preparation of solutions and rinsing. All the ILs were left open to the air for a week to achieve air equilibration before use. Synthesis of protic IL s Protic ILs, triethylammonium methylsulphonate (TAMS), EDAA and EDAF, were synthesized according to the procedure described before [36] . Briefly, the base solution (for example, triethylamine and ethylenediamine) and the acid solution (for example, methylsulphonic acid, acetic acid and formic acid) were purified, dried and handled under inert gas atmosphere. The equivalent value of neat base as well as acid was then added into the reactor simultaneously while stirred vigorously to dissipate the exothermic reaction heat. The addition rate was determined by the reaction volume and was set between 0.2 and 10 ml min −1 . The prepared protic IL samples are highly pure, as confirmed by 1 H NMR and 13 C NMR, and usually contain minimal water content in the range of ~100 p.p.m. μCP procedures Polydimethyl siloxane (PDMS) stamps were prepared from Si/SU8 masters and Sylgard 184 PDMS (Dow Corning Corporation) as per the method outlined by Whitesides et al. [11] Several different μCP strategies were tested for fabrication of IL microarray, namely indirect printing, partial printing, semi-direct printing and direct printing. Indirect printing In a typical printing experiment, ethanolic solution containing 4 mM of thiols (for example, HDT and MUA) was prepared. A PDMS stamp was inked with one drop of MUA solution for 1 min and dried gently with nitrogen stream for 30 s before printing onto a gold substrate. The gap between the patterned MUA SAM was covered by refuelling the slide with HDT. The gold slide was then rinsed twice with ethanol and dried gently with nitrogen stream. A drop of IL (for example, [BMIM][BF 4 ]) was brought into contact with the patterned area on the gold slides. The excess IL was removed by slow back suction using a micropipette. Partial printing The PDMS stamp was inked with ethanolic HDT solution and printed onto a gold substrate without refilling the gaps. The gold slide was rinsed twice with ethanol and dried with gentle nitrogen stream. A drop of IL (for example, [BMIM][BF 4 ]) was brought into contact with the patterned area on the gold slides. The excess IL was removed by slow back suction using a micropipette or by gas blowing with nitrogen. Semi-direct printing The PDMS stamp was inked with ethanolic HDT solution and printed onto a gold substrate without refilling the gaps. The gold slide was rinsed twice with ethanol and dried with gentle nitrogen stream. A drop of IL (for example, [BMIM][PF 6 ]) containing 2 mM of MUA was brought into contact with the patterned area on the gold slides. The excess IL was removed by slow back suction using a micropipette. Direct printing Microscope glass slides were first cleaned with piranha solution (3:1 concentrated H 2 SO 4 to 30% H 2 O 2 ) for 1 h (caution: this mixture reacts violently with all organic materials. The solution has to be handled with extreme care to avoid personnel injury and property damage). The slides were rinsed thoroughly with water and dried gently with N 2 stream. The preparation of organophosphanic acid SAM-modified glass surface was according to the protocol described before [15] . Briefly, PHDA monolayers were adsorbed on clean glass surfaces from 5 mM methanol solution for 12 h. The modified substrates were rinsed with methanol and dried with N 2 , and the substrates were annealed at 150 °C for 48 h under N 2 to promote stable covalent bonding formation. The annealed surfaces were then sonicated in 0.1 M K 2 CO 3 for 5 min to remove any possible multilayer and weakly bound molecules. The substrates were thoroughly rinsed with water and dried in N 2 . The PDMS stamp was inked with a droplet of IL (for example, EDAA and EDAF). Excessive IL was removed with a lint-free tissue. A thin layer of IL is formed over the PDMS and printed onto a PHDA pre-functionalized glass slide and left for 3 days. Electrochemical procedures Cyclic voltammograms were undertaken at 25±0.2 °C with a CH760 Electrochemical Workstation (CH instrument, Austin, TX, USA) in a three-electrode electrochemical cell. Gold macrodisc electrodes were used as the working electrodes. A platinum wire was used as the counter electrode and a silver or copper wire as the QRE for Ag and Cu deposition, respectively. Before measurements, the working electrodes were polished with 0.05 μm alumina slurry (CH instrument) on a clean polishing cloth (Buehler, Lake Bluff, IL, USA), sequentially rinsed with distilled water and acetone, and finally dried with lint-free tissue. The on-chip electrodeposition was carried out using the open micro-electrochemical cell configuration illustrated in Supplementary Fig. 6 . A SAM-modified gold chip fabricated by chemical vapour deposition was used as the working electrode. A Ag wire QRE and a Pt wire counter electrode were bought carefully in contact with the IL reservoirs at the edge of the IL pattern, without touching the working electrode. Controlled potential electrodeposition of Ag, Cu and AgTCNQ were performed using the gold electrode according to the procedure described before [23] , [24] , [25] . Photochemical procedures The irradiation procedure was modified from the procedure described before [37] . [BMIM][BF 4 ] solution containing 3.33 mM of AgBF 4 , 3.33 mM of TCNQ and 10% v/v of benzyl alcohol was prepared by sonication for 30 min. The IL solution was patterned onto gold surfaces and irradiated at λ =425 nm for 3 h using a Solar Simulator 50–500 W arc lamp 69907 (Newport, Stratford) coupled with a filter. Fabrication of protein microarray procedures IL solution containing 10 μM of Cyt c -OG488 or 0.75 μM of BSA–FITC and 10% v/v of phosphate-buffered saline buffer dissolution was prepared by vortexing for 5 min. The IL/protein solution was then patterned onto the gold slide via the indirect printing technique. Gas sensor experiments A gas sensor system was set up and is illustrated in Supplementary Fig. 16 . Ultra-high purity N 2 and O 2 were purchased from Air Liquide Australia (New South Wales, Australia). The flow rates and concentration of the O 2 were controlled and calculated by using four flowmeters (Cole-Palmer, New South Wales, Australia). The mixed gas was allowed to pass through a gas-mixing segment to create gas turbulence to ensure adequate mixing before entering the detection chamber. The system allows preparation of O 2 gas samples in the range from min. 130 p.p.m. to max. 100%. Amperometric gas sensing experiments were carried out using the similar electrochemical setup to metal deposition illustrated in Supplementary Fig. 6 . A hydrophobic aprotic IL, 1-n-butyl-3-methylimidazolium bistriflimide [BMIM][NTf 2 ] was patterned onto the gold macrodisc working electrode via partial printing to form 30-μm-wide IL lines with 60 μm spacing. The effective surface area of the bare gold macrodisc electrode was measured to be 0.035 cm 2 using the cyclic voltammetry method [34] . After printing, the IL covered approximately one-third of the total area of the bare gold electrode, and the effective area of electrode in contact with IL microarray was calculated to be 0.012 cm 2 . For comparison purpose, a conventional type, macroelectrode-IL gas sensor was fabricated using a gold macroelectrode of same size (0.035 cm 2 ), according to the method described in the literature [38] . Briefly, a thin layer of IL was applied to cover the gold macrodisc electrode. The thickness of the IL layer is calculated to be 100±10 μm from volume of the IL applied and the inner diameter of the electrochemical cell ( Supplementary Fig. 16 ). It should be noted that the thickness of the IL layer plays a significant role in the current responses [39] , and 100 μm thickness used in study is derived from the minimal volume of ILs that ensures a full coverage of the macroelectrode. It is also worth noting that the actual thickness of the IL layer above the electrode could be smaller than 100 μm owing to the formation of a meniscus at the edge of the cell walls. Before the experiments, the gas chamber was purged with nitrogen for 30 min to remove any traces of O 2 impurity that may presence in the systems. A constant potential of −1.2 V was applied to ensure that O 2 reduction is mass transport limited, hence all the analytes that reach the electrode will be reduced simultaneously. Under these conditions, the sensitivity of the sensor is governed mainly by the gas flow rate through the tubing, and O 2 diffusion rate from the gas phase inside the flask to the surface of the electrode [40] . Once a stable baseline was achieved, the O 2 sample was introduced into the systems. The O 2 reduction current was recorded as a function of time, and the response times were taken from the time the sensor started to respond after the gas was applied. The characteristic T 50 and T 90 values for each sensor type are measured from the time when the sensor response current reaches 50% and 90% of its steady-state value, respectively. It should be noted that response time of a gas sensor is strongly dependent on the diffusion properties of each sensor such as tubing length, flow rates, diffusion barriers and so on, and direct comparison between literatures are usually difficult [40] . Our study applied the same sensor configurations and conditions for different sensing electrode designs, which allows for sensible comparisons. Physical characterizations All reflectance micrographs were recorded using a Nikon eclipse TS100-F inverted microscope (Nikon, Japan). All phase contrast micrographs were recorded using a Nikon eclipse LV150L microscope (Nikon). Scanning confocal microscopy measurements were performed using Zeiss LSM 780 (Oberkochen, Germany). IR spectroscopy measurements were performed by Perkinelmer Spotlight 400 FTIR microscope. The recorded data were connected relative to the gold surface on reflectance mode with × 64 scan, 16 cm −1 resolution for the single-point detection. SEM measurements were performed by FEI Nova SEM 230 with a Bruker Energy Dispersive X-Ray (EDX) system operated on 10 kV accelerating voltage. The fluorescence images were taken by using a Leica DM IL LED inverted confocal microscope (Leica Microsystems, Buffalo Grove, IL, USA) or a GFP fluorescence slider (excitation filter: BP470/40, dichroic mirror: 500 and emission filter: 525/50), a mercury short-arc reflector lamp and a ProgRes CFscan camera (Jenoptik Laser, Optik, Systeme GmbH, Germany). How to cite this article: Gunawan, C. A. et al. Robust and versatile ionic liquid microarrays achieved by microcontact printing. Nat. Commun. 5:3744 doi: 10.1038/ncomms4744 (2014).